Anomalous high capacitance in a coaxial single nanowire capacitor Building entire multiple-component devices on single nanowires is a promising strategy for miniaturizing electronic applications. Here we demonstrate a single nanowire capacitor with a coaxial asymmetric Cu-Cu 2 O-C structure, fabricated using a two-step chemical reaction and vapour deposition method. The capacitance measured from a single nanowire device corresponds to ~140 μF cm −2 , exceeding previous reported values for metal–insulator–metal micro-capacitors and is more than one order of magnitude higher than what is predicted by classical electrostatics. Quantum mechanical calculations indicate that this unusually high capacitance may be attributed to a negative quantum capacitance of the dielectric–metal interface, enhanced significantly at the nanoscale. Multi-component nanowire structures in co-axial configuration, such as p-type/intrinsic/n-type silicon nanowire [1] and metal-insulator-metal (M-I-M) nanowires [2] , [3] , [4] , [5] have promising applications as fundamental building blocks in future electronic [1] , [6] , photonic [7] , power storage and delivery devices [2] , [3] , [4] , [5] . High-density and flexible capacitors are in high demand with the rapid growth of renewable energy industry. Previous work has reported values of M-I-M micro/nano-capacitors [2] , [3] , [4] , [5] with capacitance densities ranging from 2.5 to 100 μF cm −2 , via depositing alternating metallic and insulating layers inside the anodic aluminium oxide nanopores. However, such devices have high power density but low flexibility when integrating with two-dimensional architectures. This is due to the frangibility of anodic aluminum oxide templates. Whereas a direct growth of similar structures may be much easier to integrate into flexible substrate, micro/nano-electromechanical system [8] , [9] , lab-on-a-chip device [10] and so on. Here we demonstrate a single Cu-Cu 2 O-C (metal-insulator-carbon) coaxial nanowire capacitor. Cu (inner core) and C (shell) serve as conducting layers and Cu 2 O as an interfacial dielectric layer. The measured capacitance is 10–40 times larger than the value calculated based on a classic cylindered capacitor model. Remarkable capacitance density as high as 143 μF cm −2 is found for such nanowire capacitors, exceeding previously reported values of M-I-M micro/nano-capacitors [2] , [3] , [4] , [5] with capacitance densities ranging from 2.5 to 100 μF cm −2 . The Cu-Cu 2 O-C nanowires also exhibit high electrical conductivity, current-carrying capacity, as well as excellent thermal stability. Synthesis and characterization of Cu-Cu 2 O-C coaxial nanowires We use a hydrothermal reaction ( Fig. 1a,b ) to prepare PVA-coated copper nanowires templates [11] , [12] , [13] , [14] , [15] , following an annealing process that subsequently converts the copper nanowires into Cu-Cu 2 O-C coaxial structures ( Fig. 1c , Supplementary Figs S1 and S2 ). 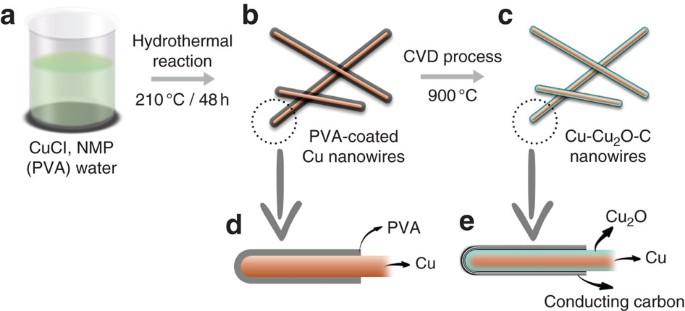Figure 1: Synthesis of Cu-Cu2O-C coaxial nanocapacitor. (a) Hydrothermal method was used to synthesize copper nanowires at 210 °C. (b) After reactions, PVA was coated on copper nanowires as the surficant, as well as the solid carbon source. The thickness of PVA can be well controlled via reaction time. (c) After annealed at 800 °C, the surface of copper nanowires will be oxidized, forming a thin cuprous oxide layer, and the PVA will carbonized to disordered graphite or amorous carbon at the outermost layer. (d) and (e) Cross-sections of PVA-coated copper nanowires before CVD process in (b) and Cu-Cu2O-C cylindrical nanocapacitor after CVD process in (c). Figure 1d and 1e illustrate the cross-sections of copper nanowires before and after the annealing process. Figure 1: Synthesis of Cu-Cu 2 O-C coaxial nanocapacitor. ( a ) Hydrothermal method was used to synthesize copper nanowires at 210 °C. ( b ) After reactions, PVA was coated on copper nanowires as the surficant, as well as the solid carbon source. The thickness of PVA can be well controlled via reaction time. ( c ) After annealed at 800 °C, the surface of copper nanowires will be oxidized, forming a thin cuprous oxide layer, and the PVA will carbonized to disordered graphite or amorous carbon at the outermost layer. ( d ) and ( e ) Cross-sections of PVA-coated copper nanowires before CVD process in ( b ) and Cu-Cu 2 O-C cylindrical nanocapacitor after CVD process in ( c ). 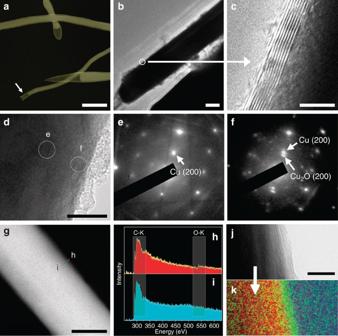Figure 2: SEM and TEM images of the coaxial structure of Cu-Cu2O-C cylindrical nanocapacitor. (a) SEM image of free-standing Cu-Cu2O-C nanowire. The carbon shell is visible in the unfilled areas (arrowed). Scale bar, 2 μm. (b) TEM image of a Cu-Cu2O-C nanowire. Scale bar, 100 nm. (c) HRTEM image taken from nanowire in (b). A seven-layer graphenic shell is visible. Scale bar, 5 nm. (d) Nano diffraction patterns from a typical nanowire. Scale bar, 20 nm. The corresponding patterns are shown in (e) and (f). The reflections from Cu2O appear close to the surface. (e) Diffraction pattern from Cu [200]. (f) Diffraction patterns from Cu [200] and Cu2O [200]. (g–i) EELS from a line scan close to the surface. Scale bar, 100 nm. (j–k) TEM image and corresponding elemental mapping the C (green) and O (red) distribution by EELS. Scale bar, 10 nm. Full size image Figure 2a is a scanning electron microscope (SEM) image of free-standing Cu-Cu 2 O-C nanowires. The cylindrical carbon layer is visible in the unfilled regions, as the white arrow marked, uniformly covering copper nanowires, whereas the interfacial thin cuprous oxide layer is difficult to see in the SEM. The carbon layers can also be identified from optical microscope images when deposited on Si/SiO 2 (285 nm) substrate ( Supplementary Fig. S3 ). Figure 2b is a transmission electron microscope (TEM) image showing the typical Cu-Cu 2 O-C nanowire. The HRTEM (high-resolution TEM image, Fig. 2c ) is taken from the circled area marked in Fig. 2b . The carbon layers in this area are graphitic and ordered, but in other areas, less-ordered graphitic or amorphous carbon shells were also seen. The interfacial insulating layer, cuprous oxide, is also clearly observed. Nano diffraction patterns ( Fig. 2d,f ) showed the presence of the Cu 2 O layer (fcc lattice). Fig. 1e shows a pattern from Cu, whereas Fig. 1f shows patterns from both Cu and Cu 2 O. The [200] reflections from both fcc lattices are marked. Figure 2g–i show EELS (extended-emission-line spectrum, electron energy-loss spectroscopy) line scans at the surface of a Cu wire. The carbon edge appears everywhere in Fig. 2i because the wire is encapsulated by a carbon shell and the sensitivity for carbon is high in EELS. Close to the surface but below the carbon shell, an oxygen edge appears in the EELS in Fig. 2h . Elemental mapping by EELS show the distribution of O and C atoms according to Fig. 2j,k , suggesting the coaxial structure of the metal-oxide-carbon architecture. Figure 2: SEM and TEM images of the coaxial structure of Cu-Cu 2 O-C cylindrical nanocapacitor. ( a ) SEM image of free-standing Cu-Cu 2 O-C nanowire. The carbon shell is visible in the unfilled areas (arrowed). Scale bar, 2 μm. ( b ) TEM image of a Cu-Cu 2 O-C nanowire. Scale bar, 100 nm. ( c ) HRTEM image taken from nanowire in ( b ). A seven-layer graphenic shell is visible. Scale bar, 5 nm. ( d ) Nano diffraction patterns from a typical nanowire. Scale bar, 20 nm. The corresponding patterns are shown in ( e ) and ( f ). The reflections from Cu 2 O appear close to the surface. ( e ) Diffraction pattern from Cu [200]. ( f ) Diffraction patterns from Cu [200] and Cu 2 O [200]. ( g–i ) EELS from a line scan close to the surface. Scale bar, 100 nm. ( j–k ) TEM image and corresponding elemental mapping the C (green) and O (red) distribution by EELS. Scale bar, 10 nm. Full size image Fabrication of Cu-Cu 2 O-C coaxial devices The fabrications of devices are illustrated in Fig. 3a,c . Cu-Cu 2 O-C coaxial nanowires were placed on number-marked SiO 2 substrates. The nanowires were partially etched by focus ion beam (FIB). Photo-lithography and e-beam evaporator were employed to pattern and deposit Cr/Au electrodes. The four-group ground-signal-ground pads are compatible for both low frequency and radio frequency measurements. 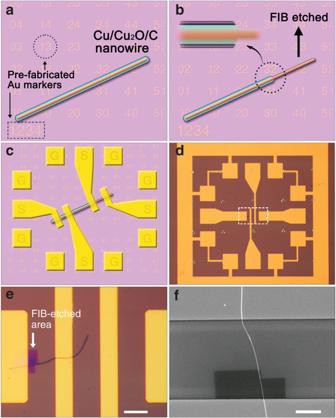Figure 3: Fabrication of Cu-Cu2O-C coaxial devices. (a) Illustration of Cu-Cu2O-C nanowires on SiO2with pre-fabricated Au markers as the arrows marked. (b) The nanowire is partially etched by FIB. Inset shows a close-up marked by the dotted circle. (c) Locate the nanowire and deposit Cr/Au signal-ground-signal (SGS) pads by photolithography. (d) Optical image of a typical device in a full view. (e) An area marked by the dotted frame in (d). The purple area marked by the arrow is etched by FIB. Scale bar, 20 μm. (f) SEM image of the nanowire. The diameter of the pristine nanowire and etched part (in black area) correspond to 130 nm and 90 nm, respectively. Scale bar, 5 μm. Figure 3d,e (dotted area in Fig. 3d ) are optical images of a fabricated Cu-Cu 2 O-C coaxial nanowire. The area in purple in Fig. 3e is etched by FIB. Figure 3f shows the corresponding SEM image indicating an outer diameter of ~130 nm and an inner diameter of ~90 nm of the coaxial nanowire. 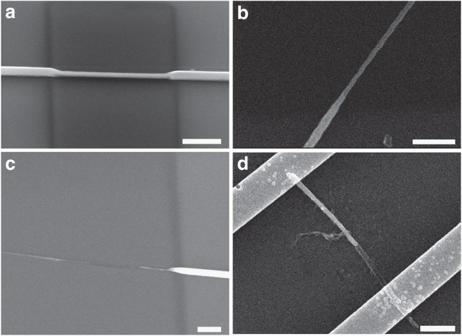Figure 4: SEM images of as-fabricated nanowires devices. (a–c) Cu-Cu2O-C coaxial nanowires were partly etched by FIB to expose the copper core. Their outer diameter and inner diameter are 120 nm, 60 nm; 100 nm, 45 nm; 80 nm, 25 nm, respectively. Scale bar, 500 nm. (d) Carbon tube device made by e-beam lithography. Scale bar, 500 nm. Figure 4a–c show Cu-Cu 2 O-C coaxial nanowires of various diameters. The minimum inner diameter can be down to ~25 nm after FIB etching ( Fig. 4c ). Figure 3: Fabrication of Cu-Cu 2 O-C coaxial devices. ( a ) Illustration of Cu-Cu 2 O-C nanowires on SiO 2 with pre-fabricated Au markers as the arrows marked. ( b ) The nanowire is partially etched by FIB. Inset shows a close-up marked by the dotted circle. ( c ) Locate the nanowire and deposit Cr/Au signal-ground-signal (SGS) pads by photolithography. ( d ) Optical image of a typical device in a full view. ( e ) An area marked by the dotted frame in ( d ). The purple area marked by the arrow is etched by FIB. Scale bar, 20 μm. ( f ) SEM image of the nanowire. The diameter of the pristine nanowire and etched part (in black area) correspond to 130 nm and 90 nm, respectively. Scale bar, 5 μm. Full size image Figure 4: SEM images of as-fabricated nanowires devices. ( a–c ) Cu-Cu 2 O-C coaxial nanowires were partly etched by FIB to expose the copper core. Their outer diameter and inner diameter are 120 nm, 60 nm; 100 nm, 45 nm; 80 nm, 25 nm, respectively. Scale bar, 500 nm. ( d ) Carbon tube device made by e-beam lithography. Scale bar, 500 nm. Full size image For control experiments, PVA tube, carbon nanotubes and pure copper nanowire devices were also prepared. The PVA tube devices can be prepared by making electrodes on the as-prepared PVA-coated copper nanowires, whereas the carbon nanotube devices could be obtained by depositing electrodes on the annealed PVA-coated copper nanowires at a high temperature ( Fig. 4e ). To obtain pure copper nanowires, the PVA layer on copper nanowires can be removed by oxygen reactive ion etching and subsequently Ar plasma to remove the possible copper oxide layer. Pure copper nanowires with a diameter of ~300 nm can also be obtained by electric deposition with anodic aluminium oxide as a template in reference samples ( Supplementary Fig. S4 ). Thermal stability of Cu-Cu 2 O-C coaxial devices Because of the excellent conductivity of the copper core and the unique coaxial structure, the Cu-Cu 2 O-C could be subjected to a current density as high as the order of 10 7 A cm −2 . Failure tests also demonstrate the excellent thermal stability of Cu-Cu 2 O-C nanowires. Even though the Cu nanowires were broken owing to a high current (>20 mA, Fig. 5a ), the carbon layers remained on the surface of copper nanowire and were clearly visible (inset in Fig. 5a ). 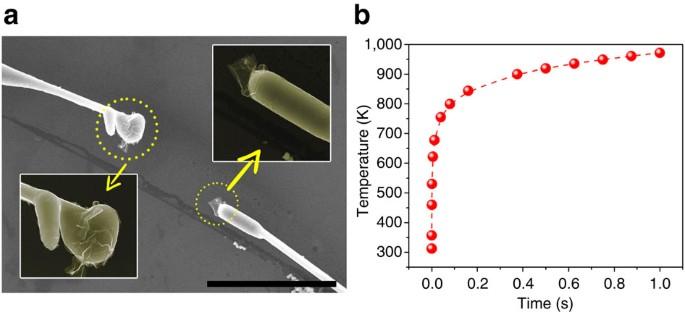Figure 5: Failure test of Cu-Cu2O-C coaxial nanowires. (a) Melting location of a broken Cu-Cu2O-C nanowire after applied a high current on it. Scale bar, 10 μm. Inset: the carbon layers remained on the surface as the arrow marked. (b) Calculated plot of temperature versus time under a high current passing the sample. Figure 5: Failure test of Cu-Cu 2 O-C coaxial nanowires. ( a ) Melting location of a broken Cu-Cu 2 O-C nanowire after applied a high current on it. Scale bar, 10 μm. Inset: the carbon layers remained on the surface as the arrow marked. ( b ) Calculated plot of temperature versus time under a high current passing the sample. Full size image The analytic expression of the temperature of the nanowire system is given by: [16] , [17] Here J and σ are current density and electric conductivity of the nanowire. w , h , and t p are the width, thickness of the nanowires and the pulse duration time, respectively. K S and μ S are the thermal conductivity and diffusivity of the substrate, respectively. The diameter, length and resistance of the nanowire ( Fig. 5a ) are ~ 600 nm, 100 μm and 29 Ω, respectively. The electrical conductivity σ and current density J are ~ 2.9×10 5 S m −1 and 7×10 10 A m −2 . The width w and thickness h of the nanowire are 600 nm. Thermal conductivity K S and diffusivity of the substrate μ S are ~30 W mK −1 and 1.2×10 −5 m 2 s −1 (aluminium oxide). The melting points can be roughly estimated at ~1000 K or even higher. According to calculations based on the heat conduction equations, the high current pulse will result in a sharp increase in temperature on the surface of the nanowires ( Fig. 5b ), suggesting that the carbon layer may work as an excellent heat shield for the whole coaxial nanowire. For comparison, I–V tests are carried out for PVA, carbon, pure copper nanowires and Cu-Cu 2 O-C nanocapacitor, respectively, as shown in Figs 6 and 7 . The resistance of PVA is ~650 MΩ ( Fig. 6a ), which is close to that of an insulator. The typical resistance of carbon nanotube and pure copper nanowire are 26.4 KΩ and 19.6 Ω ( Fig. 6b,c ), respectively. For different carbon nanotube samples, electrical conductivity ranged from 0.2×10 5 to 3.3×10 5 S m −1 , comparable to that of bulk graphite ~1.2×10 5 S m −1 (refs 18 , 19 . For the pure copper nanowires, the measured electrical conductivity ranged from 0.7×10 7 to 1.9×10 7 S m −1 , close to the value of bulk copper ~2.0×10 8 S m −1 . The conductivities of these devices are compared in Fig. 6d . I–V curves of Cu-Cu 2 O-C nanocapacitor are shown in Fig. 7a–d . For most of devices, the working voltage needs to be larger than 1 V. When a voltage less than 1 V is applied, no current could be detected (<2 pA, which can be regarded as background noise, Fig. 7a ). Although the voltage is up to 5 V, the cuprous oxide layer showed recoverable electrical breakdown ( Fig. 7b , Supplementary Fig. S5 ). The devices permanently break down if the applied voltage is large than 10 V ( Fig. 7c ) and therefore maintain a small resistance (~740 Ω, Fig. 7d ) in repeated measurements. The corresponding conductivity is ~3×10 7 S m −1 , comparable to the value from pure copper nanowires we discussed above. Such I–V behaviours can be found for most samples we have measured. According to the breakdown voltage and the typical thickness of cuprous oxide (~5–10 nm from TEM results), we estimate that the dielectric field strength of cuprous oxide is more than 100 MV m −1 , close to the value of PEFE (Teflon), a widely used insulating material in coaxial cables. 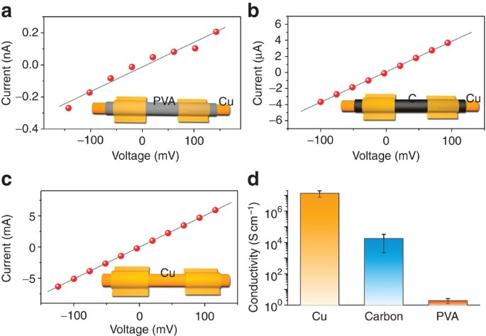Figure 6: I-V curves and conductivity of different devices. (a) PVA-coated copper nanowire. (b) Carbon-coated copper nanowire (after CVD process). (c) Pure copper nanowire. (d) Conductivity of these devices. Figure 6: I-V curves and conductivity of different devices. ( a ) PVA-coated copper nanowire. ( b ) Carbon-coated copper nanowire (after CVD process). ( c ) Pure copper nanowire. ( d ) Conductivity of these devices. 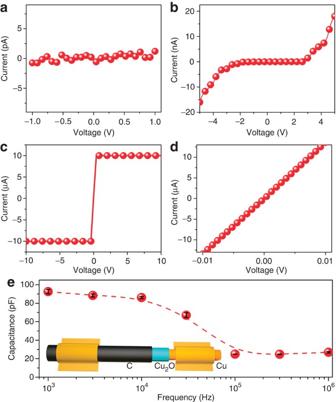Figure 7: I-V curves of voltage and frequency response of Cu-Cu2O-C cylindrical nanocapacitor (IV). (a) Voltage less than 1 V. (b) Voltage from −5 to 5 V. (c) The device is permanently broken down by applying a 10 V voltage. (d) I-V curve of Cu nanowires after breakdown of the Cu2O layer. Resistance is ~740 Ω (e) Frequency response of the device. Inset: corresponding configurations of the electrodes. Full size image Figure 7: I-V curves of voltage and frequency response of Cu-Cu 2 O-C cylindrical nanocapacitor (IV). ( a ) Voltage less than 1 V. ( b ) Voltage from −5 to 5 V. ( c ) The device is permanently broken down by applying a 10 V voltage. ( d ) I-V curve of Cu nanowires after breakdown of the Cu 2 O layer. Resistance is ~740 Ω ( e ) Frequency response of the device. Inset: corresponding configurations of the electrodes. Full size image LCR meter and network analyzer are used to study the frequency response of Cu-Cu 2 O-C nanocapacitor as shown in Fig. 7e . They have been calibrated carefully before measurements, and the noise can be suppressed down to 2fF in a wide frequency range (10 3 –10 6 Hz, Supplementary Fig. S6 ). Interestingly, for most devices, the capacitance per unit area are 28–143 μF cm −2 (at10 6 Hz), with magnitudes 10–37 times higher than that predicted by the classical electrostatics ( Supplementary Fig. S7 ). A similar result is also obtained via the radio frequency measurement ( Supplementary Fig. S8 ). These values are higher than various M-I-M capacitors built in sub-microporous templates (from 2.5 to 100 μF cm −2 ) [2] , [3] , [4] , [5] , [20] , [21] . The measured capacitance is further supported by impedance spectroscopy for Cu-Cu 2 O-C nanowires, shown in Fig. 8a . A semi circle was found in the Nyquist diagram ( Z ′ versus − Z ″, Fig. 8b ) with a red line showing the best fit, which is often found in RC circuits and is well explained based on the coaxial structure of the device. The structure of the cylindrical nanocapacitor and its equivalent circuit are illustrated in the inset of Fig. 8b . The resistance of carbon, copper core and the capacitance between them are denoted with R c , R Cu and C , respectively, as shown in the circuit. For d.c. or low frequency, current flows along the outmost graphitic layer. At high frequencies, current passes through both the graphitic layer and inner copper nanowire because the capacitance won't work at such a frequency. According to the best fit of the plot, the resistance of graphitic layer and copper core were R C ~3.2×10 5 Ω and R Cu ~30 Ω. Also, the same device measured with a DC source exhibited a resistance of ~3.5×10 5 Ω ( Supplementary Fig. S9 ), close to the fitted value. The resistance of copper nanowire core was found to be of the same order as the value for pure copper nanowires shown in Fig. 6c . The fitted capacitance between graphitic layer and copper core is ~54.9 pF, close to the value in the frequency response measurements ( Fig. 7e ). 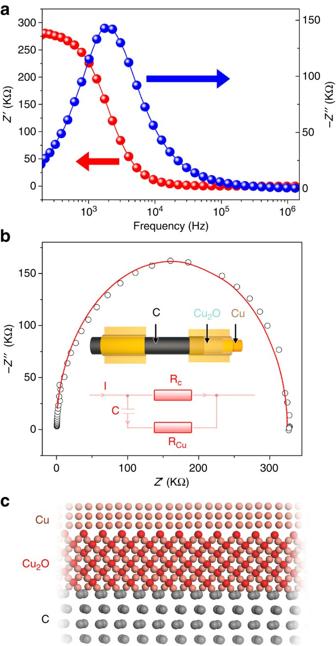Figure 8: Impedance spectra of Cu-Cu2O-C cylindrical nanocapacitors. (a) Impedance spectra of cylindrical nanocapacitor. (b)Z′ versus −Z″ fitting based on traditional cylindrical capacitor geometry.RC,RCuandCare the resistance of carbon, copper and capacitance between them, respectively. (c) Configuration of Cu-Cu2O-C capacitor [3 Cu cells-3 Cu2O cells-2 C cells] for the first-principle calculations. Figure 8: Impedance spectra of Cu-Cu 2 O-C cylindrical nanocapacitors. ( a ) Impedance spectra of cylindrical nanocapacitor. ( b ) Z ′ versus − Z ″ fitting based on traditional cylindrical capacitor geometry. R C , R Cu and C are the resistance of carbon, copper and capacitance between them, respectively. ( c ) Configuration of Cu-Cu 2 O-C capacitor [3 Cu cells-3 Cu2O cells-2 C cells] for the first-principle calculations. Full size image We have carried out detailed quantum mechanical calculations to better understand our experimental results ( Supplementary Fig. S10 and Supplementary Methods ). Figure 8c shows the configuration of Cu-Cu 2 O-C capacitor (3 Cu cells-3 Cu2O cells-2 C cells). The total capacitance of the Cu-Cu 2 O-C nanocapacitor consists of two capacitances added in series : the classical term and a quantum capacitance term. At small sizes, quantum capacitance (which is usually very large) can be the controlling factor and can either significantly decrease the effective capacitance or increase it if the quantum capacitance is negative [22] , [23] , [24] , [25] . Recent work has illustrated some interesting (and exotic) cases where negative capacitances are found, especially for oxide interfaces. Accounting for both roughness of the metal–dielectric interface and the quantum capacitance (which is indeed found to be negative for this materials system), we find that the capacitance of Cu-Cu 2 O-C capacitor can be up to 40 pF. It is important to note that quantum capacitance has such a significant effect only because of the extremely small dimensions of the dielectric. In the 5-10 nm regime (corresponding to Cu 2 O thickness), C Clas is quite high and becomes comparable to . In case of macroscopic dielectric thickness, C Clas is much smaller than and thus the latter becomes irrelevant. Our experimental process that allows fabrication of the coaxial dielectric layer at such nanoscopic dimensions provides direct experimental evidence of the significant role of quantum capacitance in nanostructures. In conclusion, we have demonstrated the synthesis and properties of a metal-insulator-carbon coaxial nanowire capacitor (Cu-Cu 2 O-C) made using a simple two-step chemical reaction and vapour deposition process. The multiple components in the structure were clearly identified by HRTEM, EELS and elemental mapping. An excellent thermal stability and remarkable capacitance were observed in individual nanowire devices. Although the gravimetric capacitance of the nanocapacitor is far less than conventional supercapacitors, [26] owing to its cylindrical structure, this nanocapacitor is a promising nanoscale coaxial cable that could be used as a transmission line for radio frequency signals at the nanoscale, as a fundamental building block in nano-architecture benefiting micro/nano-electromechanical systems and in Lab-on-a-chip type of devices [8] , [9] , [10] , [27] , [28] . Preparation of Cu-Cu 2 O-C coaxial nanowires Hydrothermal reaction ( Fig. 1a,b ) was used to prepare PVA-coated copper nanowires templates [11] , [12] , [13] , [14] , [15] , [29] . The copper source was CuCl (0.1 g, 1 mmol) mixed with an aqueous PVA solution (6 wt. %) and N -methyl-2-pyrrolidone (NMP, with a volume ratio of 1:3). They were mixed in an autoclave and react at 210 °C for 48 h. Copper nanowires coated by a PVA layer were obtained as illustrated in Fig. 1b . The thickness of PVA can be well controlled via reaction time. Shorter reaction time results in thinner PVA layers. The as-prepared PVA-coated copper nanowires were washed by distiled water and alcohol, respectively, to remove all un-reacted residues and subsequently dispersed in isopropyl alcohol. The samples solution were dropped onto SiO 2 substrate and then loaded into the centre of quartz tube for CVD (chemical vapour deposition) growth of the carbon layer [30] . The growth time is about 10 min at ~800 °C in an atmosphere of Ar/H 2 (4:1, Matheson Tri-Gas, purity: 99.999%). Higher temperature would result into a hollow carbon tube due to the evaporation of Cu. We noticed that supplying extra carbon source (CH 4 , Matheson Tri-Gas, purity: 99.99%, 10 sccm) would significantly increase the melting point of Cu nanowires. After CVD process, a thin cuprous oxide layer is found on the copper nanowires and carbon layers are formed on the outermost layer. The PVA layer acts as the oxygen source for the formation of cuprous oxide, and a solid carbon source for the carbon layer [30] , [31] , [32] as well. A thin carbon layer was formed even in absence of an external carbon source as the PVA coating layer is known to act as a solid carbon source. Fabrication of Cu-Cu 2 O-C coaxial nanocapacitors First, we dropped the as-grown Cu-Cu 2 O-C nanowires (in the isopropyl alcohol solution) on Si/SiO 2 (285 nm) substrates, where numbered Au markers have been pre-deposited for the convenience of locating the samples ( Fig. 3a ). Spin coater with a low rotation rate helped to uniformly distribute the nanowires. FIB was used to partly etch the nanowires with an optimized ion-beam dose to expose the inner Cu core ( Fig. 3b ). Typically, the nanowires will be etched with a thickness of ~30–50 nm. Next, standard photolithography or e-beam lithography processes were employed to make Cr/Au electrodes (four-group GSG pads with a size of 100×100 μm and spacer between pads is 50 μm, Fig. 3d ) on both outer shell C and inner core Cu. In detail, for photolithography, photo-resistor LOR 5B and S1813 were used to make an under-cut structure. Their thicknesses could be well controlled by adjusting the time (30–45 s) and rate (2,000–4,000 r.p.m.) of the spin coater. The electrode patterns were carefully covered on the etched nanowires using a Mask Aligner and then exposed for 4–6 s. MF319 was used to develop the photo-resistor. For e-beam lithography, PMMA was used as an e-beam resistor. JEOL 6500 was used to pattern gold electrode. The exposed sample will be developed by MIKB solution. E-beam evaporator was used to deposit Cr/Au electrode, Cr: 5 nm, Au: ~100–300 nm ( Fig. 3c ). After deposition, the devices were immersed into acetone for 24 h in room temperature to lift off the deposited metal layer. Remover PG is further used to remove the LOR 5B layer in photolithography process. Characterization and measurements A JEOL 2100F with Cs-corrected condenser was used for TEM imaging and chemical analysis. JEOL 6500F was used to characterize the morphology of samples. FEI 235 Dual-Beam Focused Ion-beam System was employed to etch Cu-Cu 2 O-C nanowires. The electrical measurements were carried out using Keithley 2400 source meters and Agilent B1500A Semiconductor Device Analyzer. The capacitance was measured by Agilent E4980A high-precision LCR meter (~20 Hz–2 MHz) and Agilent E8361C PNA Microwave Network Analyzer (~10 MHz–10 GHz, with Infinity Probes Pad pitch: 150 μm) connecting with Cascade Summit Probe Station. All the cables were connected with twisted coaxial cables. Before measurements, both devices were carefully calibrated. For LCR meter, built-in open- and short-calibrations were performed. For the network analyzer, a standard calibration was performed in a reference sample via WinCal EX program ( Supplementary Figs S6 and S8 ). How to cite this article: Liu, Z. et al . Anomalous high capacitance in a coaxial single nanowire capacitor. Nat. Commun. 3:879 doi: 10.1038/ncomms1833 (2012).